Casein kinase 2 reverses tail-independent inactivation of kinesin-1 Kinesin-1 is a plus-end microtubule-based motor, and defects in kinesin-based transport are linked to diseases including neurodegeneration. Kinesin can auto-inhibit via a head–tail interaction, but is believed to be active otherwise. Here we report a tail-independent inactivation of kinesin, reversible by the disease-relevant signalling protein, casein kinase 2 (CK2). The majority of initially active kinesin (native or tail-less) loses its ability to interact with microtubules in vitro , and CK2 reverses this inactivation (approximately fourfold) without altering kinesin's single motor properties. This activation pathway does not require motor phosphorylation, and is independent of head–tail auto-inhibition. In cultured mammalian cells, reducing CK2 expression, but not its kinase activity, decreases the force required to stall lipid droplet transport, consistent with a decreased number of active kinesin motors. Our results provide the first direct evidence of a protein kinase upregulating kinesin-based transport, and suggest a novel pathway for regulating the activity of cargo-bound kinesin. Kinesin-1 (conventional kinesin, KIF5) is an important microtubule-based molecular motor that enables fast transport towards the cell periphery. Kinesin-based transport is essential for cell function, and its impairment is linked to diseases including neurodegeneration. Discovered over two decades ago, the single molecule function of kinesin in vitro has been studied extensively, and is relatively well understood. How kinesin function is regulated in vivo , however, remains an important open question. Kinesin can auto-inhibit via a direct head–tail interaction (reviewed in ref. 1 ), but this known inhibition is released upon cargo recruitment [2] , and little is known about regulation that occurs without altering the motor's presence on cargo [3] , [4] , [5] . We report here a tail-independent inactivation for kinesin-1, reversible by casein kinase 2 (CK2). CK2 is a highly conserved, ubiquitous serine/threonine kinase important for cell growth and proliferation. There is a partial overlap in disease associations between kinesin and CK2 (tumourigenesis [6] , [7] , and neurodegeneration [8] , [9] , [10] ), but there has heretofore been no evidence of a direct functional regulatory interaction. CK2 increases the active fraction of native kinesin in vitro To probe for a potential effect of CK2 on kinesin function in vitro , we first incubated native kinesin (purified from bovine brains, Fig. 1a,b ) with recombinant CK2 holoenzyme (New England Biolabs, Fig. 1c ) in a buffer optimized for CK2 kinase activity, and then diluted the reaction (greater than tenfold) in buffer appropriate for biophysical or biochemical measurements. Parallel reactions from which CK2 had been omitted served as controls. To control for the possibility of contamination, we verified that the recombinant CK2 employed in the current study is >90% pure by Coomassie-stained SDS–PAGE gel ( Fig. 1c ), and observed no detectable contamination by mass spectroscopy ( Supplementary Table S1 ). 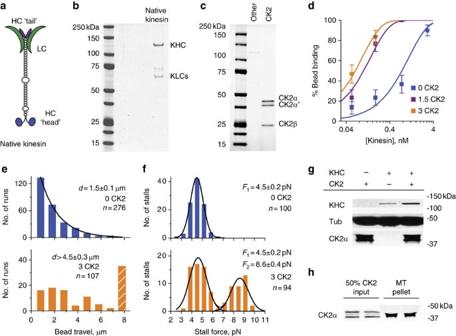Figure 1: Effect of CK2 pretreatment on native kinesin activityin vitro. Purified bovine kinesin was incubated with CK2 at 30 °C for 40 min before functional studies. '0 CK2' denotes CK2-blank samples, '1.5 CK2' (and '3 CK2') indicates an incubation ratio of 1.5 (and 3) CK2 molecules per kinesin. Values are shown as mean±s.e.m., sample sizesnare indicated. (a) Schematic of the native kinesin tetramer, including the light chains (LC) and the heavy chain (HC) 'head' and 'tail'. (b) Coomassie-stained gel of purified bovine kinesin ('Native kinesin' lane). (c) Coomassie-stained gels of recombinant human CK2 ('CK2' lane), consisting two catalytic subunits α and α′, and the non-catalytic subunit β. (d) Fraction of beads binding to microtubules at 1 mM ATP, as a function of motor concentration (each motor solution incubated with 0.6 pM 0.5 μm polystyrene beads). Beads were confined to the vicinity of microtubules with an optical trap, and 30–50 beads per trial were measured at each motor concentration. Binding fraction measurements (scatter) are well characterized by single-motor Poisson curve (solid line). A binding fraction of∼<30% indicates the single motor range11. (e) Distributions of travel distances and (f) stall forces for beads carried by kinesin(s) at 1 mM ATP. Kinesins treated with (orange) and without (blue) CK2 were compared at identical motor:bead ratios, where there was a slight contribution from a second motor for the CK2-blank sample (blue). Hatched bar in travel distribution (e) indicates travel events greater than 8 μm. The two Gaussian peaks centred at∼4.5 and∼9 pN in stall force distributions (f) correspond to one- and two-kinesin stall forces, respectively. (g) Bead-independent co-sedimentation of kinesin and CK2 with microtubules at 4 mM AMPPNP, assayed by immunoblots against tubulin ('Tub'), kinesin heavy chain ('KHC') and CK2α ('CK2α'). Relative to kinesin-blank samples, we observed a 10–19% increase in the amount of CK2 associating with microtubules in the presence of kinesin (n=2). (h) Fraction of CK2 co-sedimenting with microtubules in the absence of kinesin. Tubulin presence in the microtubule pellet lane may be visualized by its cross-reaction with the CK2α antibody. 80–85% input CK2 bound to microtubules at 4 mM AMPPNP (n=2). Figure 1: Effect of CK2 pretreatment on native kinesin activity in vitro . Purified bovine kinesin was incubated with CK2 at 30 °C for 40 min before functional studies. '0 CK2' denotes CK2-blank samples, '1.5 CK2' (and '3 CK2') indicates an incubation ratio of 1.5 (and 3) CK2 molecules per kinesin. Values are shown as mean±s.e.m., sample sizes n are indicated. ( a ) Schematic of the native kinesin tetramer, including the light chains (LC) and the heavy chain (HC) 'head' and 'tail'. ( b ) Coomassie-stained gel of purified bovine kinesin ('Native kinesin' lane). ( c ) Coomassie-stained gels of recombinant human CK2 ('CK2' lane), consisting two catalytic subunits α and α′, and the non-catalytic subunit β. ( d ) Fraction of beads binding to microtubules at 1 mM ATP, as a function of motor concentration (each motor solution incubated with 0.6 pM 0.5 μm polystyrene beads). Beads were confined to the vicinity of microtubules with an optical trap, and 30–50 beads per trial were measured at each motor concentration. Binding fraction measurements (scatter) are well characterized by single-motor Poisson curve (solid line). A binding fraction of ∼ <30% indicates the single motor range [11] . ( e ) Distributions of travel distances and ( f ) stall forces for beads carried by kinesin(s) at 1 mM ATP. Kinesins treated with (orange) and without (blue) CK2 were compared at identical motor:bead ratios, where there was a slight contribution from a second motor for the CK2-blank sample (blue). Hatched bar in travel distribution ( e ) indicates travel events greater than 8 μm. The two Gaussian peaks centred at ∼ 4.5 and ∼ 9 pN in stall force distributions ( f ) correspond to one- and two-kinesin stall forces, respectively. ( g ) Bead-independent co-sedimentation of kinesin and CK2 with microtubules at 4 mM AMPPNP, assayed by immunoblots against tubulin ('Tub'), kinesin heavy chain ('KHC') and CK2α ('CK2α'). Relative to kinesin-blank samples, we observed a 10–19% increase in the amount of CK2 associating with microtubules in the presence of kinesin ( n =2). ( h ) Fraction of CK2 co-sedimenting with microtubules in the absence of kinesin. Tubulin presence in the microtubule pellet lane may be visualized by its cross-reaction with the CK2α antibody. 80–85% input CK2 bound to microtubules at 4 mM AMPPNP ( n =2). Full size image In vitro , CK2 pretreatment significantly increased the probability of a kinesin-coated bead binding to and processing along a microtubule at 1mM ATP, in a dosage-dependent manner ( Fig. 1d ). To examine the effect of CK2 on kinesin in depth, we carried out extensive studies at a molar incubation ratio of ∼ 3 CK2 per kinesin, where effects were pronounced and approached saturation ( Fig. 1d ). Upon completion of the CK2 treatment, kinesin samples were diluted 10–1,000 times in motility buffer, and incubated with carboxylated polystyrene beads to allow for non-specific decoration of motors onto beads. Motor density on the beads was controlled by varying the input kinesin concentration, while keeping bead concentration constant. Using a conventional single beam optical trap, we positioned individual kinesin-coated beads in close vicinity of a microtubule (surface-immobilized in our flow cells) to evaluate the motor–microtubule interaction. In this confined geometry, the ability of a bead to bind to and process along the microtubule directly reflects the presence of active motors on the bead ( Supplementary Discussion ). Further, the more active motors present, the greater the probability of bead binding [11] . Remarkably, in parallel assays differing only in the presence or absence of CK2, we observed a significant enhancement in bead-binding fraction associated with CK2 treatment ( Fig. 1d ). Control experiments using beads incubated with CK2 but without kinesin showed no specific affinity to microtubules over the dilution range tested in Fig. 1d (zero bound of 50 beads tested). In the same confined geometry, CK2 treatment did not appreciably reduce the mean time between successive binding events for a bead with a single active kinesin, suggesting that the motor's 'on' rate for the microtubule was minimally affected ('Time Lapse', Supplementary Fig. S1a ). We further observed no significant effect of CK2 on the single motor travel or velocity of the active kinesin ( Supplementary Fig. S1a ), suggesting that the increase in bead-binding fraction arose from an increase in the number of active motors on the bead. To reach the single molecule range where no more than one active motor is present on the bead ( ∼ 30% binding [11] ), an additional approximately eightfold dilution was required for CK2-treated kinesin samples relative to the CK2-blank case ( Fig. 1d ). This enhancement cannot be accounted for by the minor impact of CK2 on kinesin-bead association ( Supplementary Fig. S1b, and Supplementary Methods ), thus suggesting an increase in the fraction of active motors on the bead. An increase in the active fraction of kinesins per bead is supported by two additional biophysical metrics: bead travel distance and force production. Both experimental and theoretical studies [12] , [13] demonstrate a positive correlation between cargo travel distance and motor number in vitro , and cargo force production conclusively measures the number of simultaneously engaged motors on a cargo both in vitro [14] , [15] , [16] and in vivo [4] , [5] . If CK2 does increase the active fraction of kinesins without altering its single motor function, CK2 treatment should effectively increase the number of available motors per bead, and improve both bead travel and force production. Indeed, using the same motor:bead incubation ratio where there was a small contribution from a second motor for the CK2-blank control, we observed a significant enhancement in the average bead travel (greater than threefold, Fig. 1e ) and force production (pronounced two-motor contribution at ∼ 9 pN, Fig. 1f ) associated with CK2 treatment. The unchanged one-motor peak position at ∼ 4.5 pN in force distributions ( Fig. 1f ) indicates that CK2 treatment does not alter kinesin's single motor force production. To eliminate concerns of bead-related experimental artifacts, we carried out bead-independent microtubule affinity pulldowns [17] to biochemically examine the effect of CK2 on kinesin activity. Kinesin samples (pretreated with or without CK2) were diluted tenfold in microtubule-binding buffer, and incubated with microtubules at large molar excess (>600-fold molar excess of tubulin-heterodimer to kinesin), followed by pelleting of the microtubules and associated motors. Here, AMPPNP (adenylyl imidodiphosphate, a non-hydrolysable ATP analogue) was used to increase the stability of kinesin-microtubule complexes ( Supplementary Discussion ). Consistent with the increased active motor fraction observed in the bead assay ( Fig. 1d–f , Supplementary Fig. S1a,b ), CK2 pretreatment significantly increased the fraction of native kinesin co-sedimenting with microtubules ( Fig. 1g ). This increase is unlikely to be explained by any altered interactions between the active kinesin and the microtubule: at the physiologically relevant 1 mM ATP, single-molecule biophysical measurements gave no indication of CK2 influencing either kinesin-microtubule 'on' rate or 'off' rate (as probed by time lapse between binding events, and single molecule travel distance, respectively, Supplementary Fig. S1a ). Combined, these data indicate that the effect of CK2 treatment is to increase the fraction of active kinesin molecules capable of binding to microtubules, rather than simply altering the association/dissociation rates of active kinesins with microtubules in the presence of AMPPNP. Consistent with previous reports [18] , [19] , CK2 co-sediments with microtubules with high affinity under our pulldown conditions ( Fig. 1g,h ). We observed no significant evidence of the native kinesin altering the CK2/microtubule interaction ( Fig. 1g ). The CK2 effect is independent of the kinesin tail In principle, modulation of the known head-tail binding [1] mechanism could alter the fraction of active kinesin, while leaving the single motor function intact. To conclusively test whether or not CK2 functioned by altering kinesin's head–tail interaction, we used the functional kinesin construct (K560) lacking the tail and the light chain [20] , [21] ( Fig. 2a,b ). Unless otherwise noted, a final microtubule affinity purification step [22] was used to specifically select for active K560 motors ( Fig. 2b ). We observed no detectable contamination in the microtubule-purified K560 using Coomassie-stained gels ( Fig. 2b ) or via mass spectroscopy ( Supplementary Table S1 ). The effect of CK2 pretreatment persisted for the tail-less K560, as assayed by both the bead-independent microtubule pulldowns ( Fig. 2c,d ), and the bead assays (specific or non-specific recruitment, Fig. 2e,f , Supplementary Fig. S1c,d ). Again, the single motor functions of the active K560 ( Supplementary Fig. S1c ) and K560/bead association ( Supplementary Fig. S1d ) remained unaltered, indicating that the main effect of CK2 is to increase the active motor fraction for a given K560 population. 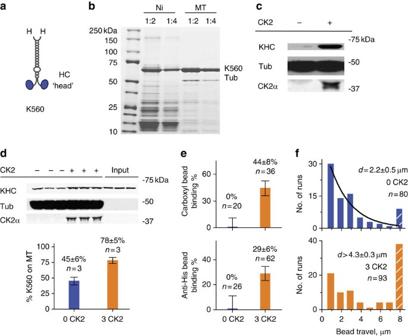Figure 2: Effect of CK2 pretreatment on K560 activityin vitro. Purified K560 was incubated with CK2 (3:1 CK2:motor) at 30 °C for 40 min (unless otherwise indicated) before functional studies. Values are shown as mean±s.e.m., sample sizesnare indicated. (a) Schematic of the tail-less kinesin, K560. Each 'H' denotes a 6xHis tag located at the C terminus of the truncated motor. (b) Purification of K560 via Ni-NTA column ('Ni'), and after a subsequent microtubule affinity pulldown and ATP release step22('MT'), assayed by Coomassie-stained gel. Two dilutions are shown (1:2 and 1:4). Microtubule affinity purification introduced some tubulin presence ('Tub') into the purified K560. (c) Bead-independent co-sedimentation of K560 and CK2 with microtubules at 4 mM AMPPNP, assayed by immunoblots against tubulin ('Tub'), kinesin heavy chain ('KHC') and CK2α ('CK2α'). (d) Co-sedimentation of freshly purified K560 with microtubules at 4 mM AMPPNP, assayed by immunoblot (top) and quantified against input motor amount (mean±s.e.m., bottom). At 2.5 h after ATP release from the final microtubule affinity purification (b), K560 was incubated with and without CK2 treatment (3:1 CK2:motor) for 1.5 h on ice and then assayed for motor activity by microtubule pulldowns. 'Input' lanes indicate the input motor amount. Approximately 55% of the initially active K560 became incapable of microtubule interaction (blue), CK2 treatment increased the active motor fraction to∼78% of input motor population (orange). (e) Bead-binding fraction measurements for both carboxyl (non-specific) and anti-His beads (specific recruitment via monoclonal antibody to C-term His-tag on K560) at 1 mM ATP (n=20–62). CK2 treatment (orange) significantly enhanced the bead-microtubule binding fraction in parallel assays. The K560:bead ratio was chosen to be sufficiently low, such that there was no measurable binding events for the CK2-blank sample (blue). For visualization sake, we graphically represent null binding with a dummy-binding fraction of 1±10%. (f) Travel distance distributions of beads moving at 1 mM ATP, compared at a K560:bead ratio where there was some contribution from a second motor in the CK2-blank control (blue). Hatched bars account for all travel events greater than 8 μm. CK2 treatment (orange) introduced a minimal twofold increase in the average bead travel. Figure 2: Effect of CK2 pretreatment on K560 activity in vitro . Purified K560 was incubated with CK2 (3:1 CK2:motor) at 30 °C for 40 min (unless otherwise indicated) before functional studies. Values are shown as mean±s.e.m., sample sizes n are indicated. ( a ) Schematic of the tail-less kinesin, K560. Each 'H' denotes a 6xHis tag located at the C terminus of the truncated motor. ( b ) Purification of K560 via Ni-NTA column ('Ni'), and after a subsequent microtubule affinity pulldown and ATP release step [22] ('MT'), assayed by Coomassie-stained gel. Two dilutions are shown (1:2 and 1:4). Microtubule affinity purification introduced some tubulin presence ('Tub') into the purified K560. ( c ) Bead-independent co-sedimentation of K560 and CK2 with microtubules at 4 mM AMPPNP, assayed by immunoblots against tubulin ('Tub'), kinesin heavy chain ('KHC') and CK2α ('CK2α'). ( d ) Co-sedimentation of freshly purified K560 with microtubules at 4 mM AMPPNP, assayed by immunoblot (top) and quantified against input motor amount (mean±s.e.m., bottom). At 2.5 h after ATP release from the final microtubule affinity purification ( b ), K560 was incubated with and without CK2 treatment (3:1 CK2:motor) for 1.5 h on ice and then assayed for motor activity by microtubule pulldowns. 'Input' lanes indicate the input motor amount. Approximately 55% of the initially active K560 became incapable of microtubule interaction (blue), CK2 treatment increased the active motor fraction to ∼ 78% of input motor population (orange). ( e ) Bead-binding fraction measurements for both carboxyl (non-specific) and anti-His beads (specific recruitment via monoclonal antibody to C-term His-tag on K560) at 1 mM ATP ( n =20–62). CK2 treatment (orange) significantly enhanced the bead-microtubule binding fraction in parallel assays. The K560:bead ratio was chosen to be sufficiently low, such that there was no measurable binding events for the CK2-blank sample (blue). For visualization sake, we graphically represent null binding with a dummy-binding fraction of 1±10%. ( f ) Travel distance distributions of beads moving at 1 mM ATP, compared at a K560:bead ratio where there was some contribution from a second motor in the CK2-blank control (blue). Hatched bars account for all travel events greater than 8 μm. CK2 treatment (orange) introduced a minimal twofold increase in the average bead travel. Full size image The CK2 effect does not require motor phosphorylation As CK2 is a kinase, we hypothesized that motor phosphorylation was responsible for CK2's effect on kinesin activity. Kinesin is an in vitro substrate for CK2 [23] , [24] , and our CK2 treatment of kinesin resulted in phosphate incorporation into both the native ( Fig. 3a ) and the tail-less motors ( Fig. 3b–e ). Focusing on tail-independent activation, via mass spectroscopy we identified one significantly phosphorylated residue in K560, a serine at 520 ( Fig. 3d , Supplementary Table S2 , and Supplementary Methods ). This serine is located in a sequence (YELLSDELN) that is a reasonable match to the CK2 phosphorylation consensus, in which acidic residues at the +1, +2 and +3 residues are important [25] . Using site-directed mutagenesis, we substituted serine 520 with alanine, and generated a functional mutant that was minimally phosphorylated by CK2 ( Fig. 3e ), suggesting serine 520 residue is indeed the main CK2 phosphorylation site in K560. Nonetheless, CK2 pretreatment still significantly enhanced the binding of this mutant kinesin to microtubules ( Fig. 3f ), indicating that phosphorylation of serine 520 is not the mechanism of CK2-mediated kinesin activation. 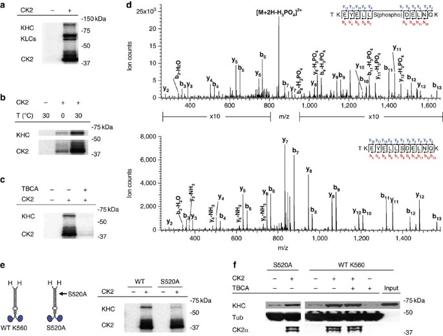Figure 3: Role of CK2 kinase activity in K560 activation. (a) Autoradiogram of CK2/native kinesin mixture, supplemented with 1 μCi of [γ-32P]-ATP. Control experiments lacking CK2 are shown. (b) Effect of incubation temperature on CK2 kinase activityin vitro, assayed by autoradiogram. Parallel samples of wild-type K560/CK2 mixture, supplemented with 1 μCi of [γ-32P]-ATP, were incubated on ice (1.5 h) or at 30 °C (40 min). Radioactive phosphate incorporation in both K560 and the CK2 itself were severely limited when incubated on ice. (c) Effect of the CK2-specific inhibitor, TBCA (100 μM), on the kinase's ability to phosphorylate wild-type K560, assayed by autoradiogram. Diminished CK2 auto-phosphorylation (in 'CK2' band) by TBCA treatment further verified the pharmacological inhibition of kinase activity. (d) LC-MS/MS spectra of tryptic phosphopeptide (TKEYELLS(phospho)DELNQK) and non-phosphopeptide (TKEYELLSDELNQK). Ion count intensity in the phosphopeptide spectrum is enhanced in the indicated regions for comparison with the non-phosphopeptide. We obtain 81% sequence coverage of K560 protein using LC-MS/MS analysis. (e) Schematic (left) of wild-type K560 and phospho-mutant S520A, and autoradiogram (right) assaying the ability of CK2 to phosphorylate the mutant ('S520A') versus wild-type motor ('WT'). (f) Motor co-sedimentation with microtubules at 4 mM AMPPNP, assayed by immunoblot. Both the phosphor-mutant ('S520A') and the wild-type motor ('WT K560') were incubated with and without CK2 (3:1 CK2:motor) for 40 min at 30 °C before microtubule pulldowns. For 'WT K560', we introduced the CK2-specific kinase inhibitor, TBCA (100 μM), during motor/kinase incubation. Figure 3: Role of CK2 kinase activity in K560 activation. ( a ) Autoradiogram of CK2/native kinesin mixture, supplemented with 1 μCi of [γ- 32 P]-ATP. Control experiments lacking CK2 are shown. ( b ) Effect of incubation temperature on CK2 kinase activity in vitro , assayed by autoradiogram. Parallel samples of wild-type K560/CK2 mixture, supplemented with 1 μCi of [γ- 32 P]-ATP, were incubated on ice (1.5 h) or at 30 °C (40 min). Radioactive phosphate incorporation in both K560 and the CK2 itself were severely limited when incubated on ice. ( c ) Effect of the CK2-specific inhibitor, TBCA (100 μM), on the kinase's ability to phosphorylate wild-type K560, assayed by autoradiogram. Diminished CK2 auto-phosphorylation (in 'CK2' band) by TBCA treatment further verified the pharmacological inhibition of kinase activity. ( d ) LC-MS/MS spectra of tryptic phosphopeptide (TKEYELLS(phospho)DELNQK) and non-phosphopeptide (TKEYELLSDELNQK). Ion count intensity in the phosphopeptide spectrum is enhanced in the indicated regions for comparison with the non-phosphopeptide. We obtain 81% sequence coverage of K560 protein using LC-MS/MS analysis. ( e ) Schematic (left) of wild-type K560 and phospho-mutant S520A, and autoradiogram (right) assaying the ability of CK2 to phosphorylate the mutant ('S520A') versus wild-type motor ('WT'). ( f ) Motor co-sedimentation with microtubules at 4 mM AMPPNP, assayed by immunoblot. Both the phosphor-mutant ('S520A') and the wild-type motor ('WT K560') were incubated with and without CK2 (3:1 CK2:motor) for 40 min at 30 °C before microtubule pulldowns. For 'WT K560', we introduced the CK2-specific kinase inhibitor, TBCA (100 μM), during motor/kinase incubation. Full size image To test the possibility that additional, less prominent phosphorylation sites might be important for the observed CK2 effect, we introduced the CK2-specific inhibitor, tetrabromocinnamic acid [26] (TBCA), to our in vitro CK2 treatment. TBCA severely limited the catalytic activity of CK2 (both motor phosphorylation and CK2 autophosphorylation, Fig. 3c ), but did not impact CK2's effects on K560 activity ( Fig. 3f ). The activation effect of CK2 on kinesin also persisted when the kinase activity of CK2 was limited by reducing the kinase/motor incubation temperature to 0°C ( Figs 2d and 3b ), again indicating that motor phosphorylation is not required for CK2 to activate K560. A non-catalytic mechanism of CK2 action is consistent with the observation that the CK2 effect is dosage dependent and approaches saturation at an incubation ratio of ∼ 3 kinases per motor ( Fig. 1d ). Co-sedimentation of CK2 with microtubules persisted after incubation with the mutant motor S520A, and was independent of CK2's kinase activity ('S520A', Fig. 3f ). The CK2 effect is specific Independent of motor phosphorylation, ice incubation of kinesin with CK2 introduced an approximately fourfold increase in the fraction of microtubule-bound motors, for both the truncated and the native kinesins ('Pre-treatment', Fig. 4a,b ). Consistent with bead assay findings ( Fig. 1b ), the activation effect of CK2 was dosage dependent, with the active fraction of the native kinesin reaching ∼ 80% of the overall motor population at 3:1 kinase:motor incubation ratio ('3CK2', Fig. 4a,b ). Control experiments using an equal molar amount of bovine serum albumin (BSA) in place of CK2 demonstrated negligible effect for both the native and the truncated kinesins ('BSA', Fig. 4a,b ). Two more independent experiments support the specificity of CK2 effect for K560. First, we verified that a different serine/threonine kinase (glycogen synthase kinase 3β, GSK3β) had no significant impact on K560 activity (3:1 GSK3β:K560, Fig. 4b ). Second, we identified differential effects of the two catalytic subunits of CK2, CK2α versus CK2α′ ( Fig. 4b ). Despite sharing 75% sequence identity [27] , the two subunits exhibited distinct effects on kinesin activity. At the same 3:1 kinase:motor incubation ratio, CK2α significantly increased the fraction of kinesin in microtubule pellets, but CK2α′ did not ( Fig. 4b ). We observed no evidence of contaminants in either subunits via Coomassie-stained SDS–PAGE gels ( Fig. 4c ). This functional specialization of CK2α versus CK2α′ again demonstrates the specificity of CK2 effect identified in the current study. 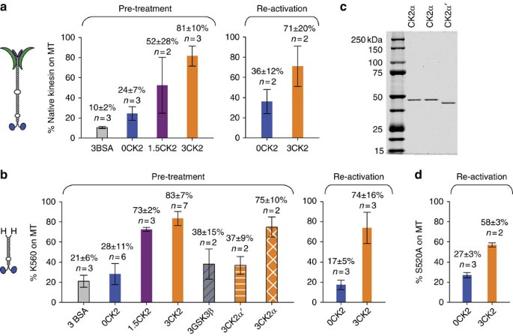Figure 4: Quantification of CK2 effect on native and truncated kinesin for both pre-treatment and re-activation. Values are shown in mean±s.e.m. for sample sizesn≥3. For sample sizen=2, values are shown in mean±data range. (a) The fraction of native kinesin capable of binding to microtubules versus input motor amount at 4 mM AMPPNP. 'Pre-treatment' and 'Re-activation' differ in their timing for microtubule pulldowns. For 'Pre-treatment', kinesin samples were incubated with CK2 or CK2-blank buffer in parallel (1.5 h on ice), followed by parallel microtubule pulldowns. Three different incubation ratios were tested: 0, 1.5 and 3 CK2 per kinesin ('0CK2', '1.5CK2' and '3CK2', respectively). Control experiments replaced CK2 with equal molar amount of BSA (3:1 BSA:kinesin, '3BSA'). For 'Re-activation', the microtubule pulldowns were staggered in time. We started with kinesin samples that were predominantly inactive ('0CK2'), and evaluated the capacity of subsequent CK2 incubation (1.5 h on ice) to reactivate these inactive kinesins ('3CK2'). We transferred the inactive kinesin to new plasticware before CK2 incubation, thus eliminating the possibility that CK2 functioned by reversing motor precipitation or adsorption to plasticware. (b) The fraction of wild-type tail-less K560 competent to bind to microtubules versus input at 4 mM AMPPNP. We employed the same 'Pre-treatment' and 'Re-activation' protocols for K560 as for the native kinesin in (a). In 'Pre-treatment', we tested the effect of various proteins in place of CK2, including using BSA (3:1 BSA:K560, '3BSA'), a different serine-threonine kinase GSK3β (3:1 kinase:K560, '3GSK3β'), and each of the two catalytic subunits of the CK2 holoenzyme (3:1 kinase:motor, '3CK2α' and '3CK2α′'). (c) Coomassie-stained gels of the two catalytic subunits of CK2: CK2α and CK2α′. Duplicate CK2α lanes are included so as not to disrupt the continuity of the gel. (d) The fraction of phospho-mutant S520A competent to bind to microtubules versus input at 4 mM AMPPNP, using the same 'Re-activation' protocol as for the native kinesin (a) and the wild-type K560 (b). Figure 4: Quantification of CK2 effect on native and truncated kinesin for both pre-treatment and re-activation. Values are shown in mean±s.e.m. for sample sizes n ≥3. For sample size n =2, values are shown in mean±data range. ( a ) The fraction of native kinesin capable of binding to microtubules versus input motor amount at 4 mM AMPPNP. 'Pre-treatment' and 'Re-activation' differ in their timing for microtubule pulldowns. For 'Pre-treatment', kinesin samples were incubated with CK2 or CK2-blank buffer in parallel (1.5 h on ice), followed by parallel microtubule pulldowns. Three different incubation ratios were tested: 0, 1.5 and 3 CK2 per kinesin ('0CK2', '1.5CK2' and '3CK2', respectively). Control experiments replaced CK2 with equal molar amount of BSA (3:1 BSA:kinesin, '3BSA'). For 'Re-activation', the microtubule pulldowns were staggered in time. We started with kinesin samples that were predominantly inactive ('0CK2'), and evaluated the capacity of subsequent CK2 incubation (1.5 h on ice) to reactivate these inactive kinesins ('3CK2'). We transferred the inactive kinesin to new plasticware before CK2 incubation, thus eliminating the possibility that CK2 functioned by reversing motor precipitation or adsorption to plasticware. ( b ) The fraction of wild-type tail-less K560 competent to bind to microtubules versus input at 4 mM AMPPNP. We employed the same 'Pre-treatment' and 'Re-activation' protocols for K560 as for the native kinesin in ( a ). In 'Pre-treatment', we tested the effect of various proteins in place of CK2, including using BSA (3:1 BSA:K560, '3BSA'), a different serine-threonine kinase GSK3β (3:1 kinase:K560, '3GSK3β'), and each of the two catalytic subunits of the CK2 holoenzyme (3:1 kinase:motor, '3CK2α' and '3CK2α′'). ( c ) Coomassie-stained gels of the two catalytic subunits of CK2: CK2α and CK2α′. Duplicate CK2α lanes are included so as not to disrupt the continuity of the gel. ( d ) The fraction of phospho-mutant S520A competent to bind to microtubules versus input at 4 mM AMPPNP, using the same 'Re-activation' protocol as for the native kinesin ( a ) and the wild-type K560 ( b ). Full size image CK2 re-activates inactive kinesin One trivial explanation for the observed CK2 effect would be that the kinase somehow prevented an irreversible inactivation of purified kinesin. As a direct test, we evaluated the effect of CK2 on already inactive kinesin ('Re-activation', Fig. 4 ). In contrast to treating kinesin with/without CK2 in parallel, before parallel microtubule pulldowns ('Pre-treatment', Fig. 4 ), in 'Re-activation' we specifically assayed for the active fraction of kinesin before and after incubation with CK2. Here, the microtubule pulldowns were staggered in time. To control for the possibility that CK2 functioned by reversing motor precipitation or adsorption onto plasticware, we transferred kinesin samples to new plasticware before CK2 incubation (so that any adsorbed motors would be left behind), and then carried out the microtubule pulldowns. Starting with samples that contained a majority of inactive motors, subsequent incubation with CK2 reversed the inactivation and resulted in a population with the majority of motors active, for both native and truncated wild-type kinesins ('Re-activation', Fig. 4a,b ), and the phospho-mutant S520A ( Fig. 4d ). These data demonstrate that tail-independent kinesin inactivation is reversible, and that the main effect of CK2 is to reverse this inactivation without requiring motor phosphorylation by the kinase. Using quantum dot (qDot) assays, we verified that CK2 could significantly increase kinesin activity after motor-qDot recruitment ( Fig. 5 ), supporting the notion that the tail-independent activation of kinesin by CK2 may in fact be feasible for cargo-bound motors. 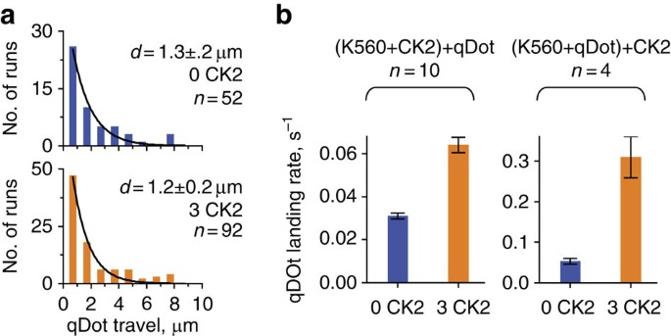Figure 5: Effect of CK2 for cargo-bound K560 assayed by qDot experiments in the single motor range. An incubation ratio of 4.3 qDot per motor was used. Values are shown as mean±s.e.m., sample sizesnare indicated. (a) Travel distributions of qDots carried by a single K560 with and without CK2 pretreatment. Purified K560 was incubated with and without CK2 (3:1 and 0:1 CK2:motor) for 1 h on ice, and then incubated with qDots (4.3:1 qDot:motor) at RT for 12 min before motility measurements. (b) Average number of motile qDots in our total internal reflection fluorescence microscope field of view (each 31x31 μm2area, 141 s observing time). We compared the effect of CK2 on kinesin activity before and after qDot recruitment. For '(K560+CK2)+qDot' (left panel,n=10 fields of view), we first incubated K560 with CK2 or CK2-blank buffer (1 h on ice), and then introduced qDots to the motor-CK2 mixture (same assay condition as ina). For '(K560+qDot)+CK2' (right panel,n=4 fields of view), we first incubated kinesin with qDots to reach a motor-qDot recruitment equilibrium (30 min on ice). Then, after this binding of K560 to the QD, we further incubated the QD-K560 complexes with CK2 or CK2-blank buffer (1 h at 4 °C). Control experiment utilizing only CK2 but not K560 did not result in any motile qDot events (or, zero landing rate). Although it is formally possible that the CK2 effect may be even more potent for cargo-bound motors, we favour the interpretation that the more pronounced enhancement of K560 activity in the '(K560+qDot)+CK2' reflects a non-linear dependence of qDot landing rate on motor-qDot ratio. Figure 5: Effect of CK2 for cargo-bound K560 assayed by qDot experiments in the single motor range. An incubation ratio of 4.3 qDot per motor was used. Values are shown as mean±s.e.m., sample sizes n are indicated. ( a ) Travel distributions of qDots carried by a single K560 with and without CK2 pretreatment. Purified K560 was incubated with and without CK2 (3:1 and 0:1 CK2:motor) for 1 h on ice, and then incubated with qDots (4.3:1 qDot:motor) at RT for 12 min before motility measurements. ( b ) Average number of motile qDots in our total internal reflection fluorescence microscope field of view (each 31x31 μm 2 area, 141 s observing time). We compared the effect of CK2 on kinesin activity before and after qDot recruitment. For '(K560+CK2)+qDot' (left panel, n =10 fields of view), we first incubated K560 with CK2 or CK2-blank buffer (1 h on ice), and then introduced qDots to the motor-CK2 mixture (same assay condition as in a ). For '(K560+qDot)+CK2' (right panel, n =4 fields of view), we first incubated kinesin with qDots to reach a motor-qDot recruitment equilibrium (30 min on ice). Then, after this binding of K560 to the QD, we further incubated the QD-K560 complexes with CK2 or CK2-blank buffer (1 h at 4 °C). Control experiment utilizing only CK2 but not K560 did not result in any motile qDot events (or, zero landing rate). Although it is formally possible that the CK2 effect may be even more potent for cargo-bound motors, we favour the interpretation that the more pronounced enhancement of K560 activity in the '(K560+qDot)+CK2' reflects a non-linear dependence of qDot landing rate on motor-qDot ratio. Full size image In vivo force depends on CK2 level but not kinase activity Might these in vitro effects be relevant in vivo ? To test this, we examined the effect of a decrease in cellular CK2α levels on cargo force production, using a lipid droplet transport system in cultured mammalian cells ( Fig. 6 ). CK2α is present on lipid droplets [28] , kinesin-1 is the predominant plus-end motor moving such droplets [4] , and the overall force driving in vivo cargos is an effective readout for the average number of engaged motors [4] , [5] . Using short interfering RNA (siRNA) transfections to specifically reduce CK2α expression in Cos-1 cells down to 12% of wild-type levels ( Fig. 6a–d , scrambled siRNA control introduced no significant effect on CK2α level), we measured a fourfold decrease in the percentage of droplets capable of escaping a fixed optical trap ('siRNA1', Fig. 6e ). Using a second siRNA to target a different region of CK2α ( Fig. 6c,d ), we observed similar reduction in cargo force production ('siRNA2', Fig. 6e ). Consistent with our finding that motor phosphorylation was not required for CK2-mediated stimulation in vitro , pharmacological inhibition of CK2 kinase activity ( Fig. 6f ) had no effect on droplet force production ('TBCA', Fig. 6e ). Significant variations in droplet size could affect force measurements, but neither knockdown of CK2α expression nor inhibition of CK2 activity had any significant effect on lipid droplet size ( Fig. 6g ). 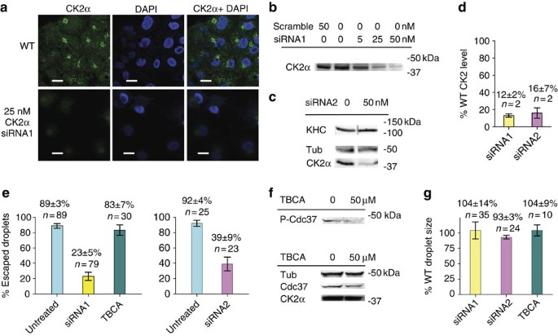Figure 6: Effect of CK2α levels and kinase activity on the number of engaged motors in cultured mammalian cells. Values are shown in mean±s.e.m. for sample sizen≥3. For sample sizen=2, values are shown in mean±data range. (a,b) Effect of siRNA treatment ('siRNA1') on CK2α level in Cos-1 cells, assayed by confocal images of immuno-fluorescence-stained Cos-1 cells (a), and by immunoblot against CK2α in cell lysates (b). Confocal images (a) were stained using 4′,6-diamidino-2-phenylindole (DAPI) and monoclonal antibody against CK2α. Control using a scrambled siRNA ('50 nM Scramble' inb) resulted in wild-type (∼98%) CK2α signal. (c) Effect of a second siRNA ('siRNA2') treatment targeting CK2α on the expression levels of CK2α and kinesin heavy chain in Cos-1 cells, assayed by immunoblot. Tubulin ('Tub') is shown as a loading control. (d) Quantitation of CK2α levels relative to the wild-type level in the two CK2α siRNA-transfected Cos-1 cells ('siRNA1', 'siRNA2'). Two distinct transfection trials were used for each siRNA. (e) Fraction of lipid droplets escaping the optical trap at a fixed laser power, in untreated wild-type (light cyan), siRNA-transfected (yellow and pink), and TBCA-treated wild-type (dark cyan) Cos-1 cells. (f) Effect of TBCA treatment (50 μM) on the kinase activity and the expression level of CK2 in wild-type Cos-1 cells, assayed by immunoblot of cell lysate. TBCA-induced reduction in CK2 kinase activity was verified by comparing the relative amount of CK2-phosphorylated form ('P-Cdc37') versus the total expression ('Cdc37') of the cell division cycle protein Cdc37 (ref.42). (g) Lipid droplet sizes in CK2α siRNA-transfected (yellow and pink) cells and TBCA-treated wild-type (dark cyan) cells relative to wild-type lipid droplet sizes. Figure 6: Effect of CK2α levels and kinase activity on the number of engaged motors in cultured mammalian cells. Values are shown in mean±s.e.m. for sample size n ≥3. For sample size n =2, values are shown in mean±data range. ( a , b ) Effect of siRNA treatment ('siRNA1') on CK2α level in Cos-1 cells, assayed by confocal images of immuno-fluorescence-stained Cos-1 cells ( a ), and by immunoblot against CK2α in cell lysates ( b ). Confocal images ( a ) were stained using 4′,6-diamidino-2-phenylindole (DAPI) and monoclonal antibody against CK2α. Control using a scrambled siRNA ('50 nM Scramble' in b ) resulted in wild-type ( ∼ 98%) CK2α signal. ( c ) Effect of a second siRNA ('siRNA2') treatment targeting CK2α on the expression levels of CK2α and kinesin heavy chain in Cos-1 cells, assayed by immunoblot. Tubulin ('Tub') is shown as a loading control. ( d ) Quantitation of CK2α levels relative to the wild-type level in the two CK2α siRNA-transfected Cos-1 cells ('siRNA1', 'siRNA2'). Two distinct transfection trials were used for each siRNA. ( e ) Fraction of lipid droplets escaping the optical trap at a fixed laser power, in untreated wild-type (light cyan), siRNA-transfected (yellow and pink), and TBCA-treated wild-type (dark cyan) Cos-1 cells. ( f ) Effect of TBCA treatment (50 μM) on the kinase activity and the expression level of CK2 in wild-type Cos-1 cells, assayed by immunoblot of cell lysate. TBCA-induced reduction in CK2 kinase activity was verified by comparing the relative amount of CK2-phosphorylated form ('P-Cdc37') versus the total expression ('Cdc37') of the cell division cycle protein Cdc37 (ref. 42 ). ( g ) Lipid droplet sizes in CK2α siRNA-transfected (yellow and pink) cells and TBCA-treated wild-type (dark cyan) cells relative to wild-type lipid droplet sizes. Full size image Tail-independent inactivation occurs for monomeric kinesin What is the mechanism responsible for the tail-independent kinesin inactivation? One possibility is that kinesin might form oligomers and thereby become inactive. To address this, we utilized size-exclusion chromatography to investigate potential changes in kinesin sizing profile before and after inactivation ( Supplementary Methods ). The K560 peak location did not change ( Fig. 7a ), but the associated motor activity was significantly reduced (approximately fivefold, assayed by the bead-binding fraction, Fig. 7b ). This result suggests that protein aggregation is not important for the reversible kinesin inactivation observed in the current study. A second possibility is that the 'inactive' kinesin state might occur when the motor binds to ADP, given that the equilibrium binding of kinesin to microtubules has been reported to be weak for ADP-bound motors [29] , [30] ( K d ∼ 10–20 μM). Using dialysis (80 mM pipes pH 7.0, 5 mM ETDA, Supplementary Methods ) to deplete potential bound nucleotides in Ni-purified K560, we again observed significant loss of motor activity for the dialysed K560 after ice incubation ('Dialysed', 'Before' versus 'After', Fig. 7c ). Although the completeness of dialysis-mediated nucleotide removal was difficult to assess, the fraction of K560 capable of binding to microtubules remained the same as for the un-dialysed samples ('Undialysed, after', Fig. 7c ) and for the dialysed samples where ADP was introduced back in ('Dialysed+ADP, after', Fig. 7c ) that underwent identical ice incubation. Thus, kinesin inactivation is unlikely to simply reflect ADP binding. A third possibility is that there might be an inhibitory head–head interaction, which could block the microtubule binding of the kinesin dimers. To test this, we generated a truncated kinesin (K339) that exists as a functional monomer [31] . For this K339 monomer, motor inactivation still persisted and was again rescued by CK2 ( Fig. 7d ). Therefore, the tail-independent kinesin inactivation identified in the current study cannot require head–head interaction. Based on these findings, we hypothesize that the tail-independent kinesin inactivation may involve a conformational change within individual kinesin heads, at least somewhat independent of their nucleotide-bound states. 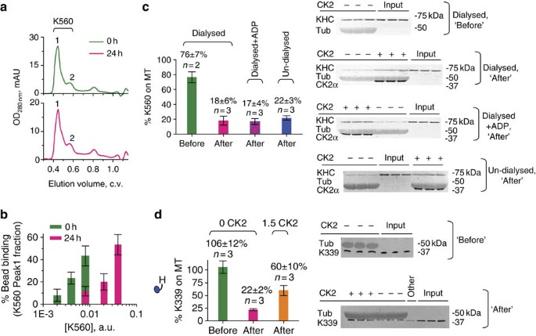Figure 7: Mechanism studies of K560 inactivation. Values are mean±s.e.m., sample sizesnare indicated. (a,b) Role of oligomerization. The oligomerization state (a) and activity (b) of K560 immediately after Ni purification (0 h), and after a 24 h ice incubation (24 h). (a) Size exclusion chromatography using Superdex-200. K560 content was verified by Coomassie (not shown) and bead assay (b). Peak positions 1 and 2 were well correlated with the dimeric and monomeric forms of Eg5-513-GFP analysed using the same column43. Relative abundance of peak 1 versus 2 was 4.73±0.86 at 0 h, and 4.4±0.43 at 24 h (mean±data range,n=2 each). (b) Motor activity in peak 1 elute, analysed by bead assay (n∼30) at 1 mM ATP. When compared at the same motor concentration per bead, approximately fivefold less K560 dilution was required to reach the same bead binding fraction at the 0th h. (c) Role of nucleotide-bound state. The fraction of K560 competent for microtubule binding at 4 mM AMPPNP, before and after a 1.5 h incubation on ice, assayed by immunoblot against kinesin heavy chain (AKIN01). Cross reactivity of the polyclonal antibody AKIN01 with tubulin ('Tub') is used for loading control. Input reference lanes are as indicated ('Inputs'). Ni-purified K560 was dialysed against 5 mM EDTA to deplete bound nucleotide, and then supplemented with 10 mM Mg2+('Dialysed') or 10 mM Mg2+/10 mM ADP ('Dialysed+ADP'). Controls used un-dialysed K560 undergoing identical ice incubation ('Un-dialysed'). The effect of CK2 during incubation is quantified later in the text. We hypothesize that an additional freeze-thaw cycle may contribute to the increased magnitude of inactivation observed in (c) versus (b). (d) Role of head–head interaction. Co-sedimentation of K339 monomer (C-term His-tagged, 'H') with microtubules at 4 mM AMPPNP, assayed by immunoblot against kinesin heavy chain (AKIN01). Cross reactivity of AKIN01 with tubulin ('Tub') was used for loading control. Shown are microtubule pulldowns using Ni-purified K339 immediately after thawing ('Before'), or after incubation with or without CK2 (1.5:1 kinase:monomer) for 1.5 h on ice ('After'). Input reference lanes are as indicated ('Inputs'). The lane marked as 'Other' (in 'After' immunoblot,d) was not part of the current study. Figure 7: Mechanism studies of K560 inactivation. Values are mean±s.e.m., sample sizes n are indicated. ( a , b ) Role of oligomerization. The oligomerization state ( a ) and activity ( b ) of K560 immediately after Ni purification (0 h), and after a 24 h ice incubation (24 h). ( a ) Size exclusion chromatography using Superdex-200. K560 content was verified by Coomassie (not shown) and bead assay ( b ). Peak positions 1 and 2 were well correlated with the dimeric and monomeric forms of Eg5-513-GFP analysed using the same column [43] . Relative abundance of peak 1 versus 2 was 4.73±0.86 at 0 h, and 4.4±0.43 at 24 h (mean±data range, n =2 each). ( b ) Motor activity in peak 1 elute, analysed by bead assay ( n ∼ 30) at 1 mM ATP. When compared at the same motor concentration per bead, approximately fivefold less K560 dilution was required to reach the same bead binding fraction at the 0th h. ( c ) Role of nucleotide-bound state. The fraction of K560 competent for microtubule binding at 4 mM AMPPNP, before and after a 1.5 h incubation on ice, assayed by immunoblot against kinesin heavy chain (AKIN01). Cross reactivity of the polyclonal antibody AKIN01 with tubulin ('Tub') is used for loading control. Input reference lanes are as indicated ('Inputs'). Ni-purified K560 was dialysed against 5 mM EDTA to deplete bound nucleotide, and then supplemented with 10 mM Mg 2+ ('Dialysed') or 10 mM Mg 2+ /10 mM ADP ('Dialysed+ADP'). Controls used un-dialysed K560 undergoing identical ice incubation ('Un-dialysed'). The effect of CK2 during incubation is quantified later in the text. We hypothesize that an additional freeze-thaw cycle may contribute to the increased magnitude of inactivation observed in ( c ) versus ( b ). ( d ) Role of head–head interaction. Co-sedimentation of K339 monomer (C-term His-tagged, 'H') with microtubules at 4 mM AMPPNP, assayed by immunoblot against kinesin heavy chain (AKIN01). Cross reactivity of AKIN01 with tubulin ('Tub') was used for loading control. Shown are microtubule pulldowns using Ni-purified K339 immediately after thawing ('Before'), or after incubation with or without CK2 (1.5:1 kinase:monomer) for 1.5 h on ice ('After'). Input reference lanes are as indicated ('Inputs'). The lane marked as 'Other' (in 'After' immunoblot, d ) was not part of the current study. Full size image CK2 effect is mediated by weak K560/kinase interaction Thus far, our data indicate that neither the kinesin tail ( Figs 2 , 3 , 4 , 5 ) nor phosphorylation ( Figs 3 and 4d ) is required for CK2-mediated kinesin activation. Using immunoprecipitation assays ( Supplementary Methods ) against kinesin's carboxy terminal (C-terminal) His tag ( Fig. 8a ) or heavy chain ( Fig. 8b ), we observed complex formation/co-immunoprecipitation between CK2 and K560, independent of CK2's kinase activity. Intriguingly, when tested separately, of the two catalytic subunits, only CK2α′ co-immunoprecipitated with K560 ( Fig. 8b ). Nonetheless, CK2α—but not CK2α′—demonstrated similar potency for kinesin activation as the CK2 holoenzyme (immunoblot for one of two trials shown in Fig. 8c , quantified in Fig. 4b ). We conclude from these data that the functional interaction between CK2 and the tail-less kinesin is specific but weak. Immunofluorescence staining of untreated wild-type Cos-1 cells demonstrated some co-localization between CK2α and kinesin heavy chain ( Fig. 8d,e , Supplementary Methods ), and provides support for the likelihood of a weak interaction in vivo . We note that there appeared to be cell-to-cell variation in the amount of co-localization of CK2 and kinesin, as judged either by eye or the cross-correlation analysis. Thus, we suspect that the CK2–kinesin interaction may be regulated, and may be an interesting topic for future studies. 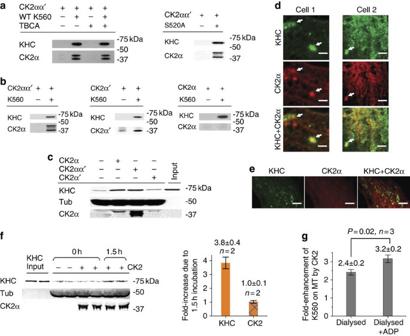Figure 8: Mechanism of CK2-mediated activation. (a) Role of motor phosphorylation in motor/kinase interaction (co-immunoprecipitation against the motor's His-tag). Equal molar ratio of the untagged CK2 holoenzyme and K560 (with or without TBCA) or S520 was used. (b) Role of CK2 subunits in motor/kinase interaction (co-immunoprecipitation using SUK4 against the KHC (kinesin heavy chain)). K560 was incubated in equal molar ratio with CK2αα′ (holoenzyme), CK2α′, or CK2α. (c) Functional effects of CK2 subunits versus holoenzyme (all at 3:1 kinase:motor ratio, 1.5 h on ice) on K560 activity, assayed by microtubule pulldowns at 4 mM AMPPNP. Microtubule-bound kinesin increased due to CK2 holoenzyme and CK2α treatment, but not CK2α′; one of two trials shown. (d,e) Spatial correlation between KHC and CK2α in TIRF imaged Cos-1 cells, stained against kinesin heavy chain (SUK4) and CK2α. Scale bars, 2 μm. (d) Representative cytosolic areas from two cells. Arrows highlight local overlap between CK2α and KHC signals. 66±1% of kinesin detected co-localized with CK2α (mean±s.e.m.,n=3). Control analysis using uncorrelated images between cell 1 and 2 gave a baseline value of 33±6% (mean±data range,n=2). (e) A third Cos-1 cell. KHC signal was in general rather punctate, somewhat different from the more diffuse distribution of CK2α. (f) Importance of initial interaction between K560 and CK2, before exposure to microtubules, assayed by microtubule pulldowns at 4 mM AMPPNP. Starting with K560 samples that were predominantly inactive ('−', '0 h'), we evaluated the ability of CK2 (3:1 kinase:motor) to reactivate K560 with and without extended incubation/interaction with the motor before adding the microtubules ('+', '1.5 h' versus '0 h'). The increase in microtubule-bound K560 due to the 1.5 h incubation, shown in immunoblot (left panel), is quantified (relative to the 0 h time point) in the bar graph (right panel, mean±data range,n=2). (g) Fold enhancement of microtubule-bound motors, for K560 in the nucleotide-free ('Dialysed') and the ADP-bound states ('Dialysed+ADP'). K560 used in dialysis experiments was not specifically selected for motor activity, may explain the more modest CK2 effect.P-value was evaluated usingt-test. Values are shown as mean±s.e.m., using results from three independent dialysis experiments. Figure 8: Mechanism of CK2-mediated activation. ( a ) Role of motor phosphorylation in motor/kinase interaction (co-immunoprecipitation against the motor's His-tag). Equal molar ratio of the untagged CK2 holoenzyme and K560 (with or without TBCA) or S520 was used. ( b ) Role of CK2 subunits in motor/kinase interaction (co-immunoprecipitation using SUK4 against the KHC (kinesin heavy chain)). K560 was incubated in equal molar ratio with CK2αα′ (holoenzyme), CK2α′, or CK2α. ( c ) Functional effects of CK2 subunits versus holoenzyme (all at 3:1 kinase:motor ratio, 1.5 h on ice) on K560 activity, assayed by microtubule pulldowns at 4 mM AMPPNP. Microtubule-bound kinesin increased due to CK2 holoenzyme and CK2α treatment, but not CK2α′; one of two trials shown. ( d , e ) Spatial correlation between KHC and CK2α in TIRF imaged Cos-1 cells, stained against kinesin heavy chain (SUK4) and CK2α. Scale bars, 2 μm. ( d ) Representative cytosolic areas from two cells. Arrows highlight local overlap between CK2α and KHC signals. 66±1% of kinesin detected co-localized with CK2α (mean±s.e.m., n =3). Control analysis using uncorrelated images between cell 1 and 2 gave a baseline value of 33±6% (mean±data range, n =2). ( e ) A third Cos-1 cell. KHC signal was in general rather punctate, somewhat different from the more diffuse distribution of CK2α. ( f ) Importance of initial interaction between K560 and CK2, before exposure to microtubules, assayed by microtubule pulldowns at 4 mM AMPPNP. Starting with K560 samples that were predominantly inactive ('−', '0 h'), we evaluated the ability of CK2 (3:1 kinase:motor) to reactivate K560 with and without extended incubation/interaction with the motor before adding the microtubules ('+', '1.5 h' versus '0 h'). The increase in microtubule-bound K560 due to the 1.5 h incubation, shown in immunoblot (left panel), is quantified (relative to the 0 h time point) in the bar graph (right panel, mean±data range, n =2). ( g ) Fold enhancement of microtubule-bound motors, for K560 in the nucleotide-free ('Dialysed') and the ADP-bound states ('Dialysed+ADP'). K560 used in dialysis experiments was not specifically selected for motor activity, may explain the more modest CK2 effect. P -value was evaluated using t -test. Values are shown as mean±s.e.m., using results from three independent dialysis experiments. Full size image Under our microtubule pulldown conditions, CK2 exhibited strong interaction with microtubules ( Fig. 1h ). In principle, CK2 might function simply by acting as a microtubule-associated protein that recruited kinesin to the microtubule, and an initial kinesin–CK2 interaction might not be relevant. To test this possibility, we prepared identical CK2/K560 mixtures (3:1 kinase:motor), and evaluated the importance of a 1.5 h incubation of CK2 with kinesin before introducing microtubules ( Fig. 8f ). Here, the same amount of CK2, K560 and microtubules were used, and microtubule pulldown assay conditions were identical (that is, the mixture of CK2 and K560 was in the presence of the microtubules for the same amount of time). We observed a significant increase in K560 activity only for samples that had undergone extended incubation with the kinase ( Fig. 8f ) before being exposed to microtubules. However, CK2 binding to microtubules was not affected by the motor/kinase incubation, and there was no increase in the amount of CK2 on the MTs correlating with the ∼ 3.8-fold increase in kinesin activity ( Fig. 8f ). These data indicate that an initial functional interaction between CK2 and K560 is necessary, and a model where CK2 first binds to MTs, and then recruits kinesin, is inconsistent with our data. However, we cannot rule out other contributions of the microtubule to this process (see below). Although CK2 and kinesin co-immunoprecipitate in vitro , the presence of kinesin did not enhance the fraction of CK2 binding to microtubules ( Fig. 1g ). We hypothesize that CK2 may have a stronger binding to the microtubule than to the K560. This possibility might provide a mechanism for dissociating the CK2/kinesin complex after functional interaction. Activation effect of CK2 is enhanced for ADP-bound kinesins The hypothesized CK2-mediated alteration in kinesin conformation (within individual motor heads), coupled with the weak interaction between kinesin and CK2 ( Fig. 8g ), suggests that an additional change occurs to drive the motor activation. Although kinesin's inactivation itself may not depend on ADP presence, part of the CK2-mediated activation process could involve a change in kinesin's nucleotide-bound state. To test this, we returned to the dialysed K560 motors that approximates the motor's nucleotide-free state ('Dialysed', quantified in Fig. 8g , immunoblot for one dialysis trial shown in Fig. 7c ), and tested whether CK2's ability to activate kinesin was affected when we introduced ADP back into the dialysed sample ('Dialysed+ADP', quantified in Fig. 8g , immunoblot for one dialysis trial shown in Fig. 7c ). Intriguingly, CK2 was able to activate kinesin more effectively when ADP was present ( Figs 7c and 8g ). Additionally, when ADP was present in the dialysed sample, the effect of CK2 approached that for the un-dialysed samples (54±4% versus 67±10%, respectively, mean±s.e.m., n =3 trials each, immunoblots for one dialysis trial shown in Fig. 7c ), and we observed no significant impact of additional ADP on CK2 effect in un-dialysed kinesin samples (data not shown). The exact sensitivity of the CK2 effect to ADP may in fact be larger, depending on the completeness of nucleotide depletion in dialysis. Nonetheless, the observed difference is statistically significant ( P =0.02, t -test, Fig. 8g ), tested for three independent dialysis trials (immunoblot for one of three trials shown in Fig. 7c ), and is consistent with the hypothesis that ADP binding/release may contribute to the activation process. Additional possibilities include conformation changes in CK2 as a result of motor binding, or competition between microtubules and K560 for CK2 binding. Complete mechanistic details remain to be investigated in future studies. Taken together, our data uncovers a tail-independent inactivation for kinesin-1, reversible by CK2. Although other members of the kinesin family may have modes of regulation in addition to the tail-mediated auto-inhibition [32] , this is the first evidence to our knowledge of a second regulatory mode for kinesin-1. When tested with freshly purified K560 that was specifically selected for motor activity (via microtubule affinity purification step [22] , Fig. 2b ), the time scale of this tail-independent inactivation and re-activation ( ∼ 4 h and 1.5 h, respectively, Supplementary Discussion ) was significantly faster than the turn-over rate of the native kinesin in vivo (half-life of 18–20 h [33] ). Inactivation/activation could occur more rapidly; our temporal resolution is limited by assay conditions including motor-kinase incubation. The finding that kinase activity of CK2 was not required for kinesin activation was unexpected. However, there are precedents: kinase-independent regulation has been reported for CK2 affecting microtubules [19] and other kinases/targets [34] , [35] , [36] . It remains possible that phosphorylation by CK2 might serve as an intermediate state for additional kinases [37] to enable further spatial and/or temporal regulation of the kinesin motor. The tail-independent activation of kinesin identified here suggests a novel pathway for cell signalling to reversibly regulate kinesin activity, while the motors remain cargo associated. A recent report demonstrates that the number of engaged motors is actively regulated during axonal transport, even though the overall motor presence on cargo remains constant [3] . Other regulatory pathways could also take advantage of this activation pathway, either by blocking access of CK2 to the kinesin (to promote inactivation) or alternatively, by directly interacting with kinesin and mimicking the CK2 effect. As kinesin activation is tuned by CK2 levels ( Figs 1d and 4a,b ), changes in cellular CK2 concentration likely lead to corresponding changes in kinesin activity. This is consistent with live cell force measurements ( Fig. 6 ), and suggests the possibility of a link between CK2 enrichment [38] and the preferential recruitment of kinesin to microtubules in the initial segment of axons [39] . Our study also suggests an intriguing role for altered CK2 signalling [7] , [8] , [10] in disease progression: by influencing transport processes crucial for cell function. The extent to which this occurs for both neurodegenerative diseases (where CK2 is often decreased and transport likely impaired) and cancers (where CK2 is increased and transport is likely unregulated to support metastasis) remains an exciting area for future research. Proteins Native kinesin and tubulin were purified from bovine brain [15] , [40] . Functional tail-less K560 (refs 20 , 21 ), monomer K339 (ref. 31 ), and phospho-mutant S520A were constructed using plasmid pET17b_k560 (ref. 20 ) (Addgene) as template. Protein was bacterially expressed and Ni-NTA purified [21] . To specifically select for motor activity, unless otherwise noted Ni-eluted K560 was further purified by microtubule affinity purification [22] before flash freezing in 10% sucrose and storage at −80 °C. Human recombinant CK2 holoenzyme (CK2αα′, un-tagged), CK2α and GSK3β (both C-terminal His-tagged), and CK2α′ (amino terminal His-tagged) were purchased from New England Biolabs, Invitrogen and Millipore, respectively. The same activation effects for kinesin were observed for three different lots of CK2 holoenzyme tested (NEB, Lot 0130802, 0140810, 14/021309). Immunoblot Primary antibodies used were SUK4 and tubulin-α (Developmental Studies Hybridoma Bank, University of Iowa), AKIN01 (Cytoskeleton), CK2α (Cell Signaling) and CK2α′ (Novus Biologicals). For immunoblots, primary antibody concentrations used were: 1:500 for SUK4; 1:300–500 for tubulin-α; and 1:1,000 for AKIN01, CK2α and CK2α′. Immunoblots were quantified using Odyssey (Li-Cor Biosciences). In vitro CK2 pre-treatment 75 nM purified kinesin (native or truncated) was incubated with recombinant CK2 (holoenzyme or subunit as indicated, up to 250 nM, New England Biolabs) in 20 μl reaction buffer (20 mM tris–HCl pH 7.5, 50 mM KCl, 10 mM MgCl 2 , 0.5 mM EGTA, plus 500 μM ATP) at 30 °C for 40 min (optimal for CK2 kinase activity), or 0 °C for 1.5 h. Reactions from which CK2 had been omitted served as controls. To block CK2 kinase activity, 100 μM CK2-specific inhibitor TBCA [26] (EMD Chemicals, Inc.) was introduced to above assays, with ethanol as a control. For functional characterizations (bead and qDot assay, microtubule pulldown), samples were placed on ice after allotted incubation time without further quenching of CK2 kinase activity. To assay for phosphate incorporation, motor/kinase reaction (0.5 μg kinesins per 250U CK2, 30 °C for 40 min as suggested by the manufacturer) were supplemented with 1 μCi of [γ- 32 P]-ATP (Perkin Elmer), quenched with reducing SDS sample buffer, separated by SDS–PAGE, and visualized by PhosphorImager (Amersham). In vitro CK2 re-activation CK2-blank kinesins (thawed, 150 nM native or truncated dimer, or 300 nM monomer) were first incubated on ice for 1.5 h. This ice incubation does not impact the active fraction of native kinesin ( ∼ 20% immediately after thawing), but significantly reduces the active fraction of truncated kinesins (dimer or monomer, down to ∼ 20%). After ice incubation, 10 μl each of the kinesin samples are identically transferred to two sets of new Eppendorf tubes. For one set, 10 μl CK2-blank reaction buffer was added, followed immediately by a microtubule pulldown assay to determine the active motor fraction. For the second set containing identical kinesin samples, 10 μl CK2 (500 nM) was added, followed by a 1.5 h kinase:motor incubation on ice, then assayed for active motor fraction via microtubule pulldown. Microtubule affinity pulldown Kinesin (20 μl of 75 nM native or truncated dimer or 150 nM monomer, with indicated amounts of CK2 holoenzyme or subunit, and indicated incubation conditions) were incubated with microtubule-binding solution (180 μl containing 5 μM microtubule, 80 mM Pipes pH 6.9, 50 mM CH 3 CO 2 K, 4 mM MgSO 4 , 1 mM DTT, 1 mM EGTA, 20 μM taxol), supplemented with 4 mM AMPPNP (EMD), for 15 min at room temperature (RT). The reaction was centrifuged in a TLS55 rotor for 10 min at 170,000 g at 25 °C. The resulting microtubule pellet was dissolved in 30 μl 1× reducing SDS sample buffer, separated by SDS–PAGE, and analysed by immunoblot. Addition of 1 mg ml −1 casein in the microtubule-binding solution did not alter CK2-mediated kinesin activation. In vitro optical trap Kinesin was first incubated with CK2 (75 nM native or K560, indicated CK2 amount and conditions), then titrated and incubated with 0.6 pM carboxylated polystyrene beads (0.5 μm, Polysciences) in 100 μl motility buffer (80 mM Pipes pH 6.9, 50 mM CH 3 CO 2 K, 4 mM MgSO 4 , 1 mM DTT, 1 mM EGTA, 10 μM taxol, 1 mg ml −1 casein) for 15 min at RT for non-specific recruitment. Here, bead concentration was chosen to optimize the number of beads in our field of view, and was kept constant while we varied kinesin concentration (up to ∼ 2,000-fold dilution starting from 75 nM) to vary motor:bead incubation ratio, and thereby control motor presence on individual beads. In case of K560, we also used anti-His beads [41] (0.4 μm) to specifically recruit the motor via its C-terminal His-tag. Anti-His beads [41] were prepared by incubating 20 μl penta-His biotin conjugate (Qiagen) with 10 μl streptavidin-coated polystyrene beads (1% solids, Spherotech) in 100 μl 1×PEM80 buffer for 30 min at 4 °C, and washed five times in 1×PEM80 buffer containing 8 mg ml −1 BSA or 5.55 mg ml −1 casein before use. K560 concentration was titrated after indicated treatment (starting at 75 nM) and incubated with 1 μl anti-His beads in total 15 μl motility buffer for 15 min at RT. After incubation, motor-bead mixture were flown into flowcells with preassembled microtubules [15] , and all measurements were carried out at RT in motility buffer, supplemented with 1 mM ATP, and an oxygen-scavenging system (250 μg ml −1 glucose oxidase, 30 μg ml −1 catalase, 4.5 mg ml −1 glucose). Bead-microtubule binding was tested using an optical trap ( K trap ∼ 0.005 pN nm −1 ) to position each bead near a microtubule. A binding event is scored if the bead processes away from the trap within a wait time of 30 s. Extending wait times to 2 min had no effect on binding fraction measured (see Supplementary Discussion ). Bead force production was monitored by the bead positions in the trap ( K trap =0.0436±0.001 pN nm −1 ). Bead motility was measured with trap turned off upon a binding event. Where appropriate, travel distributions were fitted to a single exponential decay to extract the characteristic run length and associated uncertainties. For measurements where CK2 treatment significantly increased the population exceeding our 8-μm field view, algorithmic mean (and associated error) was used to determine the minimum average travel and associated error. Stall force distributions were fitted to Gaussians to extract mean one- and two-motor forces, and the associated errors. Error on binding fractions ( p ) was determined as , for n beads tested. In vitro quantum dot Quantum dots (QDots) (qDot-655 Carboxyl, Invitrogen) were excited with 488 nm laser (Ti:Sapphire, Coherent) and imaged via a custom total internal reflection fluorescence microscope (Nikon 1.49NA, ×100), recorded at 4.25 fps (Photmetrics Quantem 512SC). Motility assays utilized the same motility buffer and flow chamber (with preassembled microtubules) as for bead assays, and analysis was carried out using a custom-tracking program (Gross Lab) that identifies qDot positions via 2D Gaussian fitting of their brightness profile. For CK2 pretreatment, K560 was first incubated with CK2 (75 nM K560, 0 or 250 nM CK2, 1 h on ice), then diluted (25-fold) to incubate with qDots at 4.3:1 qDot:motor ratio in 6 μl motility buffer for 12 min at RT. The reaction was then brought up to 20 μl in motility buffer, supplemented with 1 mM ATP and oxygen-scavenging system, followed by motility experiments. For CK2 effect on motors already in complex with qDot, 75 nM K560 was first incubated with qDots at 4.3:1 qDot:motor ratio in 6 μl moltility buffer for 30 min at 4 °C. The kinesin/qDot mixture was then divided into equal 3 μl portions and incubated with 3 μl each of 0 or 250 nM CK2 for 1 h at 4 °C. The reaction was then diluted (35-fold) in motility buffer, and 20 μl each was supplemented with 1 mM ATP and an oxygen-scavenging system, followed by motility experiments. Cell culture and CK2α knockdown Cos-1 cells were grown in DMEM (Invitrogen) supplemented with 10% fetal bovine serum at 37 °C in 5% CO 2 . Gene silencing was achieved by transfection with two different commercially available CK2α siRNAs, from Qiagen (with sense strand 5′-CAUUGAAGCUGAAAUGGUATT-3′) and Santa Cruz Biotechnology, Inc (a pool of three different siRNA duplexes with sense strands 5′-GAAGCCAUCAACAUCACAATT-3′, 5′-GAUCCACGUUUCAAUGAUATT-3′ and 5′-CCUCAGUCUUGUAAAUGUATT-3′), using the Hiperfect transfection reagent and according to manufacturer's instructions. Non-silencing siRNA and non-transfected cells were included as controls. The final dosing concentration of all siRNAs provided was 50 nM, unless otherwise noted, and the cells were incubated with the siRNA transfection complexes for 24 h in complete media at normal growth conditions. After 24 h in complete media at normal growth conditions (additional 50 μM TBCA in growth media for TBCA treatment), the cells were treated with 60 μg ml −1 of fatty acid-albumin complex to induce the lipid droplet formation. The cells were then exposed to DMEM without glucose and fatty acid for 16 h, before immediate lipid droplet-trapping experiments. For cell lysates, scrapped-off cells were washed with PBS and lysed in ice-cold lysis buffer (25 mM Tris–HCl pH 7.5, 150 mM NaCl, 1% NP40, 1 mM EDTA, 1 mM PMSF, 1 mM Na 3 VO 4 , and 1× protease inhibitor cocktail). Live cell escape force measurements Lipid droplets in Cos-1 cells were visualized by differential interference contrast microscopy, the force driving individual lipid droplets was determined by monitoring the droplet motion inside an optical trap [4] , [5] . An escape event was scored if the droplet moved out of the optical trap within the 30 s wait period. A no-escape event was scored if the trapped droplet could not escape the trap, but resumed motion once the trap was turned off. We empirically tuned the trap power (980 nm, 24 mW output) such that the majority ( ∼ 80–90%) of lipid droplets in wild-type cells could escape the trap, and measured escape events for all cells under the same trap power for direct comparison. Droplet sizes were manually quantified in ImageJ. Errors in escaped fraction ( f ) were determined as , for n droplets tested. How to cite this article: Xu, J. et al . Casein kinase 2 reverses tail-independent inactivation of kinesin-1. Nat. Commun. 3:754 doi: 10.1038/ncomms1760 (2012).